Dynamin−SNARE interactions controltrans-SNARE formation in intracellular membrane fusion The fundamental processes of membrane fission and fusion determine size and copy numbers of intracellular organelles. Although SNARE proteins and tethering complexes mediate intracellular membrane fusion, fission requires the presence of dynamin or dynamin-related proteins. Here we study these reactions in native yeast vacuoles and find that the yeast dynamin homologue Vps1 is not only an essential part of the fission machinery, but also controls membrane fusion by generating an active Q a SNARE-tethering complex pool, which is essential for trans -SNARE formation. Our findings provide new insight into the role of dynamins in membrane fusion by directly acting on SNARE proteins. Both size and copy number of intracellular organelles can alter in reproducible ways upon changes in environmental conditions or in response to the cell cycle. Examples of these organelles include endosomes, lysosomes, vacuoles and mitochondria [1] , [2] , [3] . Critical for the determination of the organelle size is the magnitude of ongoing fusion and fission reactions, which must be tightly regulated. Membrane fusion in the endomembrane system involves cognate sets of v- (vesicular or R) and t- (target or Q a , Q b and Q c ) SNAREs. SNAREs from two fusing membranes form trans -complexes between the membranes [4] , [5] , [6] , [7] . Many tethers, like the vacuolar homotypic fusion and vacuole protein sorting (HOPS) complex, physically interact with SNAREs and may stimulate the formation of trans -SNARE complexes by bringing the opposing membranes in closer contact [8] , [9] . In addition to tethering complexes, many other proteins have been identified to interact with SNAREs, including Munc13, V-ATPase, dynamins, complexins, synaptotagmins and Sec1/Munc18 proteins [10] , [11] . How these proteins help to coordinate the SNARE-mediated fusion process with the antagonistic membrane fission reaction is an area that has remained unexplored. It is not clear whether the fission machinery for different organelles is related, or fission occurs in unique, organelle-specific ways. One potential common factor is dynamin-like GTPases, which are important for vacuolar and mitochondrial fission [2] , [3] . Under suitable conditions, dynamins form spiral- or ring-like collars on artificial liposomes, leading to their tubulation and fragmentation upon GTP hydrolysis [12] , [13] , [14] . The GTPase effector domain and the middle domain of dynamin have been shown to be needed for self-assembly and allosteric regulation of the GTPase activity [13] , [15] . Interestingly, recent studies have revealed the involvement of dynamin in granular exocytosis [16] . In an earlier study, we showed a dual function of the dynamin-like protein, Vps1, in membrane fission and fusion [17] ; however, the underlying molecular mechanism allowing Vps1 to regulate both processes has remained unexplored. Here we investigate the molecular mechanism of how Vps1 controls membrane fusion and coordinates fusion with the antagonistic fission process. Vps1 controls trans -SNARE formation Vacuoles purified from vps1Δ strains are fusion incompetent [17] . In contrast to pure vps1Δ fusions, mixed fusions employing wild-type and vps1Δ vacuoles displayed considerable fusion activity (~50% of wild-type levels, Fig. 1a ). Fusion efficiency was determined by measuring alkaline phosphatase activity; pro-alkaline phosphatase in the BJ vacuoles is activated by maturation enzymes contained in DKY vacuoles [17] . As trans -SNARE complex formation is essential for successful fusion, we asked first whether the absence of trans -SNARE formation accounts for the fusion defect of vps1Δ vacuoles. Yeast vacuoles harbour four SNAREs that are required for their fusion [18] . The Q a SNARE Vam3, the Q b SNARE Vti1, the Q c SNARE Vam7 and the R-SNARE Nyv1 form the trans -SNARE complexes necessary for fusion. A characteristic feature of vacuolar fusion is its homotypic architecture, meaning that both fusion partners harbour the same SNARE composition on their respective surfaces [18] . To analyse the trans -SNARE complex formation, we tagged either Nyv1 or Vam3 on wild-type and vps1Δ vacuoles. Addition of the haemagglutinin (HA) or vesicular stomatitis virus (VSV) tag to the carboxy terminus did not impair SNARE function ( Supplementary Fig. S1A ). Priming and docking occur in the presence of ATP. Accordingly, no trans -SNARE interactions were detectible in the absence of ATP. When Vam3-HA was precipitated from wild-type vacuoles in the presence of ATP, Nyv1-VSV co-precipitated from wild-type vacuoles, indicating that normal trans -SNARE formation had occurred ( Fig. 1a ). However, when Vam3-HA was precipitated from vps1Δ vacuoles, no co-precipitating Nyv1-VSV could be detected, suggesting that Vps1 might be an essential factor for successful trans -SNARE formation. 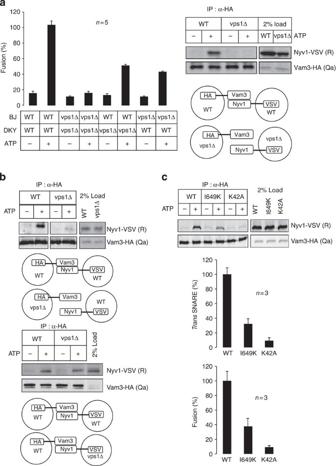Figure 1: Vps1 controlstrans-SNARE formation. (a) Vacuoles derived from wild-type (BJ and DKY) andvps1Δ (BJ and DKY) strains were incubated under standard fusion condition. Mixed fusions containing wild-type andvps1Δ vacuoles displayed 50% fusion activity when compared with pure wild-type fusions. Five independent experiments are shown as means±s.d. Vacuoles harbouring either Vam3-HA or Nyv1-VSV were isolated from wild-type andvps1Δ yeast cells.Trans-SNARE assays were performed as described in the Methods section. Vacuoles purified fromvps1Δ vacuoles do not establishtrans-SNAREs. (b) Vacuoles harbouring either Vam3-HA or Nyv1-VSV were isolated from wild-type andvps1Δ yeast cells.Trans-SNARE assays were performed as mentioned in the Methods section. In the top panel,trans-SNARE formation of Vam3-HA-tagged vacuoles derived from wild-typeor vps1Δ strains with Nyv1-VSV-tagged vacuoles purified from wild-type cells are displayed. In the bottom panel, Vam3-HA tagged vacuoles from wild-type cells were mixed with wild-type orvps1Δvacuoles harbouring Nyv1-VSV. Onvps1Δ vacuoles, only the QaSNARE Vam3 but not the R-SNARE Nyv1 is impaired in its capability to enter intotrans-SNARE complexes. (c) Vacuoles purified from wild-type, I649K and K42A strains harbouring Vam3-HA or Nyv1-VSV were examined fortrans-SNARE complex formation. Means±s.d. of three independent experiments are shown. Vacuoles purified from wild-type, I649K and K42A strains were examined for fusion activity as described in the Methods section. Three independent experiments are shown as means±s.d. Figure 1: Vps1 controls trans -SNARE formation. ( a ) Vacuoles derived from wild-type (BJ and DKY) and vps1 Δ (BJ and DKY) strains were incubated under standard fusion condition. Mixed fusions containing wild-type and vps1 Δ vacuoles displayed 50% fusion activity when compared with pure wild-type fusions. Five independent experiments are shown as means±s.d. Vacuoles harbouring either Vam3-HA or Nyv1-VSV were isolated from wild-type and vps1 Δ yeast cells. Trans -SNARE assays were performed as described in the Methods section. Vacuoles purified from vps1 Δ vacuoles do not establish trans -SNAREs. ( b ) Vacuoles harbouring either Vam3-HA or Nyv1-VSV were isolated from wild-type and vps1 Δ yeast cells. Trans -SNARE assays were performed as mentioned in the Methods section. In the top panel, trans -SNARE formation of Vam3-HA-tagged vacuoles derived from wild-type or vps1 Δ strains with Nyv1-VSV-tagged vacuoles purified from wild-type cells are displayed. In the bottom panel, Vam3-HA tagged vacuoles from wild-type cells were mixed with wild-type or vps1Δ vacuoles harbouring Nyv1-VSV. On vps1 Δ vacuoles, only the Q a SNARE Vam3 but not the R-SNARE Nyv1 is impaired in its capability to enter into trans -SNARE complexes. ( c ) Vacuoles purified from wild-type, I649K and K42A strains harbouring Vam3-HA or Nyv1-VSV were examined for trans- SNARE complex formation. Means±s.d. of three independent experiments are shown. Vacuoles purified from wild-type, I649K and K42A strains were examined for fusion activity as described in the Methods section. Three independent experiments are shown as means±s.d. Full size image An earlier study showed that Vps1 controls Vam3 function [17] . Moreover, mixed fusions between wild-type and vps1Δ vacuoles retained 50% of fusion activity ( Fig. 1a ), suggesting that not all SNAREs are functionally affected by the vps1Δ mutation. Therefore, we asked what topology of trans -SNARE complex formation might account for the mixed fusion array. Again, when Vam3-HA was precipitated from wild-type vacuoles upon addition of ATP, Nyv1-VSV co-precipitated from wild-type vacuoles, indicating that normal trans -SNARE formation had occurred ( Fig. 1b , top panel). However, when Vam3-HA was originating from vps1Δ vacuoles, Nyv1-VSV did not co-precipitate even from wild-type vacuoles ( Fig. 1b , top panel). Another picture emerged when Vam3-HA was precipitated from wild-type vacuoles. In this case, Nyv1-VSV from wild-type or vps1Δ vacuoles was able to interact in trans with Vam3-HA from wild-type vacuoles ( Fig. 1b , bottom panel). These data suggest that the vps1Δ phenotype does not lead to a general disability of all vacuolar SNAREs, but specifically hits the Q a SNARE Vam3 in its function to enter into trans -SNARE complexes, further confirming the role of Vps1 in controlling Vam3 activity during membrane fusion. Next we tested whether point mutations in Vps1 might confer defects on vacuolar fusion and the trans -SNARE complex formation. The K42A mutation leads to a GTP-hydrolysis-defective Vps1 protein [19] , [20] , [21] and the I649 mutation affects the self-assembly of Vps1 ( [22] , [23] ; Supplementary Fig. S1B ). Vacuoles purified from these strains exhibited dramatically reduced fusion activity and, concomitantly, little or no trans -SNARE complex formation ( Fig. 1c ). These data suggest that the amount of trans -SNARE complex formation is directly connected to the physical state of Vps1. To promote efficient trans -SNARE formation, Vps1 needs to hydrolyse GTP and has to be present in a polymeric state. The interaction of the Q a SNARE Vam3 with HOPS requires Vps1 To further elucidate the molecular impact of Vps1 mutations on the function of Vam3 in vacuolar fusion and trans -SNARE establishment, we investigated the abundance of different Vam3 pools on wild-type and vps1Δ vacuoles. Vam3 can reside in different states on the vacuolar surface, either as a single SNARE bound to the tethering complex HOPS or interacting with the NSF/Sec18 adapter protein Sec17/α-SNAP and other SNAREs as part of vacuolar cis -SNARE complexes [24] . We selectively precipitated Sec17 and Vps33 from detergent-extracted wild-type and vps1Δ vacuoles using antibodies specific for Sec17 or the HA extension of Vps33. Vps33 is the vacuolar SM protein and an integral part of the HOPS complex [25] . Addition of the HA extension to the C terminus did not impair Vps33 function ( Supplementary Fig. S2 ). We found Vps1 to be significantly enriched in the Vps33-HA fraction precipitated from wild-type detergent extracts and almost totally absent in the Sec17 pulldown ( Fig. 2a ). A significantly lower level of Vam3 co-precipitated with Vps33-HA in vps1Δ vacuoles when compared with wild-type Vps33-HA precipitations, although the total amount of precipitated Vps33 was almost equal ( Fig. 2a ). However, the amount of Vam3 associated with Sec17 in vps1Δ vacuoles was comparable to wild-type levels. This suggests that only in the presence of Vps1, Vam3 is able to interact with the HOPS complex and is not exclusively found in Sec17-associated cis -SNARE complexes ( Fig. 2a ). SNAREs must interact with the tethering complex HOPS to establish trans- SNARE complexes [25] , [26] , [27] . We found that Vam3 is associated with the HOPS complex and Vps1 ( Fig. 2b ). However, the composition of this complex was changed upon addition of ATP. When Vps33-HA was precipitated from wild-type vacuoles in the presence of ATP, Vps1 was released from the Vam3–HOPS complex ( Fig. 2b ). Most likely, this reaction is controlled by NSF/Sec18, as temperature inactivation of this ATPase led to impaired release activity of Vps1 from the Vam3–HOPS complex ( Supplementary Fig. S3 ). On the basis of the observation that Vps1 controls SNARE–HOPS associations and trans -SNARE formation, we determined whether mutations in Vps1 might affect these interactions. We measured the Q a -SNARE density on the HOPS complex by precipitating Vps33-HA from wild-type and mutant vacuoles. Interestingly, we detected a correlation between the extent of Vam3–HOPS coprecipitation rates and fusion efficiency ( Figs. 2c , 1c ). Whereas the K42A mutant exhibited rates much like the vps1Δ strain, the I649K mutant showed about 35% of the wild-type Vam3– coprecipitation signal, which matched the fusion efficiency of this mutant ( Figs. 2c , 1c ) when compared with wild type. 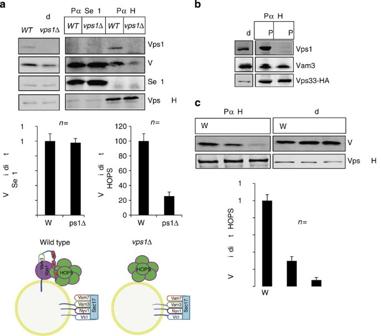Figure 2: The interaction of Vam3 with HOPS requires Vps1. (a) Wild-type andvps1Δvacuoles were detergent extracted and immunoprecipitated either with anti Sec17 antibodies or with anti HA antibodies. Immunoprecipitation assay was done as explained in the Methods section. Vam3 binding to Sec17 and Vam3 binding to Vps33-HA were quantified using Odyssey software. Means±s.d. of three independent experiments are shown. The diagrammatic model displays the different Vam3-containing complexes on wild-type andvps1Δvacuoles. (b) Vps1 is released from HOPS-Vam3 in the presence of ATP. Wild-type vacuoles were incubated for 15 min in the absence and presence of ATP. After detergent extraction, Vps33-HA was precipitated and co-precipitating proteins were analysed by western blotting. (c) Vacuoles purified from wild-type, K42A and I649K strains were processed as described inb. Vps33-HA was precipitated from detergent extracts and co-precipitating proteins were analysed. The band intensity was quantified from three independent experiments. Means±s.d. of three independent experiments are shown. Figure 2: The interaction of Vam3 with HOPS requires Vps1. ( a ) Wild-type and vps1Δ vacuoles were detergent extracted and immunoprecipitated either with anti Sec17 antibodies or with anti HA antibodies. Immunoprecipitation assay was done as explained in the Methods section. Vam3 binding to Sec17 and Vam3 binding to Vps33-HA were quantified using Odyssey software. Means±s.d. of three independent experiments are shown. The diagrammatic model displays the different Vam3-containing complexes on wild-type and vps1Δ vacuoles. ( b ) Vps1 is released from HOPS-Vam3 in the presence of ATP. Wild-type vacuoles were incubated for 15 min in the absence and presence of ATP. After detergent extraction, Vps33-HA was precipitated and co-precipitating proteins were analysed by western blotting. ( c ) Vacuoles purified from wild-type, K42A and I649K strains were processed as described in b . Vps33-HA was precipitated from detergent extracts and co-precipitating proteins were analysed. The band intensity was quantified from three independent experiments. Means±s.d. of three independent experiments are shown. Full size image Vps1 specifically binds to the Vam3 SNARE domain As the release activity of Vps1 from Vam3 is a prerequisite [17] for successful vacuolar fusion ( Fig. 2b ), we asked, whether the addition of excess rVps1 might compensate for the release of endogenous Vps1 from Vam3, and hence might inhibit vacuolar fusion. We confirmed this by adding an increasing amount of rVps1 to fusion reactions (IC 50 ~1.8 μM, Fig. 3a and Supplementary Fig. S4 ) and, moreover, addition of rVps1 (5 μM) to vacuoles completely suppressed trans -SNARE formation ( Fig. 3b ). 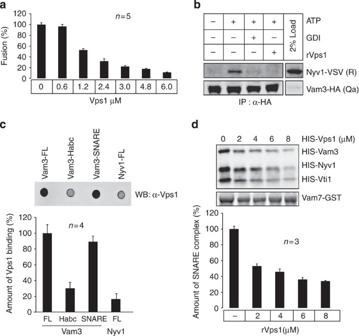Figure 3: Vps1 specifically binds to the QaSNARE Vam3. (a) Recombinant Vps1 inhibits vacuole fusion. Vacuoles derived from BJ3505 and DKY6805 strains were incubated with increasing concentration of rVps1 in standard fusion reaction as described in the Methods section. Vacuolar fusion was completely inhibited at a concentration of 6 μM rVps1. (b) Recombinant Vps1 inhibitstrans-SNARE formation. Thetrans-SNARE assay was performed as described. Recombinant Vps1 was added to the assay at a concentration of 6 μM. GDI, which extracts the small G-protein Ypt7 from the vacuolar membrane, was added as an inhibitor oftrans-SNARE formation at a concentration of 5 μM. At the given concentration, rVps1 suppressedtrans-SNARE formation much like GDI. (c) Vps1 binds to the SNARE domain of Vam3. 1 μg of full-length Vam3, N-terminal domain of Vam3 (1–190), SNARE domain of Vam3 (190–252) and full-length Nyv1 were immobilized on a nitrocellulose membrane and incubated with rVps1 overnight. Detection of bound rVps1 was performed as described in the Methods section. Means±s.d. of three independent experiments are shown. Only full-length Vam3 and the SNARE domain of Vam3 displayed binding towards rVps1. (d) Recombinant Vps1 inhibits SNARE complex formation. The indicated recombinant proteins (2 μg for all SNAREs) were incubated with increasing concentrations of rVps1 for 1 h at 4 °C and subsequently Vam7-GST was precipitated. Co-precipitating proteins were analysed using SDS–PAGE and western blotting. In the presence of 6 μM rVps1, SNARE complex formation is suppressed up to 65%. Three independent experiments are shown as means±s.d. Figure 3: Vps1 specifically binds to the Q a SNARE Vam3. ( a ) Recombinant Vps1 inhibits vacuole fusion. Vacuoles derived from BJ3505 and DKY6805 strains were incubated with increasing concentration of rVps1 in standard fusion reaction as described in the Methods section. Vacuolar fusion was completely inhibited at a concentration of 6 μM rVps1. ( b ) Recombinant Vps1 inhibits trans -SNARE formation. The trans -SNARE assay was performed as described. Recombinant Vps1 was added to the assay at a concentration of 6 μM. GDI, which extracts the small G-protein Ypt7 from the vacuolar membrane, was added as an inhibitor of trans -SNARE formation at a concentration of 5 μM. At the given concentration, rVps1 suppressed trans -SNARE formation much like GDI. ( c ) Vps1 binds to the SNARE domain of Vam3. 1 μg of full-length Vam3, N-terminal domain of Vam3 (1–190), SNARE domain of Vam3 (190–252) and full-length Nyv1 were immobilized on a nitrocellulose membrane and incubated with rVps1 overnight. Detection of bound rVps1 was performed as described in the Methods section. Means±s.d. of three independent experiments are shown. Only full-length Vam3 and the SNARE domain of Vam3 displayed binding towards rVps1. ( d ) Recombinant Vps1 inhibits SNARE complex formation. The indicated recombinant proteins (2 μg for all SNAREs) were incubated with increasing concentrations of rVps1 for 1 h at 4 °C and subsequently Vam7-GST was precipitated. Co-precipitating proteins were analysed using SDS–PAGE and western blotting. In the presence of 6 μM rVps1, SNARE complex formation is suppressed up to 65%. Three independent experiments are shown as means±s.d. Full size image Having established that Vps1 controls Vam3 function during the trans -SNARE formation ( Fig. 1b ), we sought for an experimental approach, which would allow us to convincingly demonstrate the specificity of Vps1 binding towards Vam3. In addition, we were interested in what domain of Vam3 might interact with Vps1. We therefore performed dot blot experiments by immobilizing full-length Vam3, the amino-terminal Habc domain, the SNARE domain of Vam3 and full-length Nyv1 onto nitrocellulose membranes. When the immobilized proteins were exposed to rVps1, only full-length Vam3 and the SNARE domain of Vam3 exhibited binding towards Vps1 ( Fig. 3c ). We determined the Kd of Vam3–Vps1 interactions by biolayer interferometry using an Octet Red 96 instrument (ForteBio Inc.) at 3.63 × 10 −7 M ( Supplementary Fig. S5 ). To confirm that Vps1 mainly interacts with the SNARE domain of Vam3, we investigated the SNARE complex formation of recombinantly expressed SNAREs in the presence of increasing concentrations of rVps1 ( Fig. 3d ). We speculated that Vps1 might sequester Vam3 from the SNARE complex, leading to decreased numbers of tetrameric SNARE complexes. Indeed, in the presence of rVps1, SNARE complex formation was suppressed up to 65% ( Fig. 3d ). Dynasore inhibits vacuolar fission and fusion in vivo Yeast vacuoles fragment upon cellular exposure to hypertonic stress [17] or at the onset of bud emergence [3] as visualized by fluorescence microscopy after staining with the fluorescent dye FM4-64 [17] . Using the hypertonic stress response, we visualized the inhibition of vacuolar fission and fusion in vivo by dynasore. Dynasore is a small molecule, selective non-competitive inhibitor of the protein dynamin [28] . Logarithmic-phase yeast cells were stained with FM4-64. To first explore the effect of dynasore on vacuolar fission, we added either dynasore or the solvent dimethylsulphoxide (DMSO) to the stained cells and subsequently induced fission by a brief high-salt exposure ( Fig. 4A , upper panel). DMSO did not inhibit vacuolar fragmentation as visualized by the increased number of smaller vacuoles (70% of vacuoles fragmented; Fig. 4A upper panel), whereas dynasore diminished this amount drastically (only 20% of vacuoles fragmented; Fig. 4A upper panel). To assess the in vivo effect of dynasore on vacuolar fusion, we fragmented the stained vacuoles by brief salt exposure and subsequently added dynasore or DMSO ( Fig. 4A , lower panel). After release of the vacuoles from the hypertonic media, vacuoles started to refuse, but this was significantly less efficient in the presence of dynasore (only 50% of the DMSO control, Fig. 4A , lower panel). Along with our in vivo investigations, we confirmed the inhibitory effect of dynasore on vacuole fusion and trans -SNARE formation in vitro . In the presence of 100 μM dynasore, we could not observe any trans -SNAREs formation and vacuolar fusion ( Fig. 4B ). The GTPase activity of rVps1 was inhibited up to 60% by dynasore ( Fig. 4C ). These data indicate that Vps1 function is critical for controlling vacuolar fission and fusion. 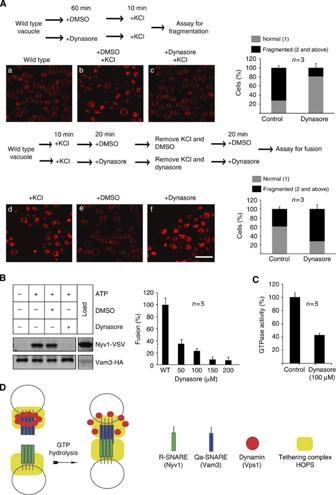Figure 4: Dynasore inhibits vacuolar fission and fusionin vivo. (A) Vacuoles of wild-type yeast cells were labelled with FM4-64 using the standard procedure as described in the Methods section. In the assay for fragmentation, (a) shows the normal vacuole structure of logarithmic phase wild-type cells, (b) shows salt-induced fragmentation of vacuoles in the presence of solvent DMSO. (c) Salt-induced phenotype of vacuoles in the presence of 100 μM dynasore. The percentage of cells showing normal or fragmented vacuoles was quantified. One hundred cells were counted randomly in each experiment. Three independent experiments are shown as means±s.d. In the assay for fusion (d) shows the fragmented vacuoles after salt exposure; (e) shows the effect of the solvent DMSO on re-fusion of fragmented vacuoles; (f) displays the influence of dynasore on re-fusion of fragmented vacuoles. The percentage of cells exhibiting normal or fragmented vacuoles was quantified. One hundred cells were counted randomly in each experiment. Three independent experiments are shown as means ±s.d. Scale bar 5 μm. (B) Dynasore at a concentration of 100 μM inhibitsin vitrovacuole fusion andtrans-SNARE complex formation. (C) Dynasore inhibits the GTPase activity of recombinant Vps1. (D) Model explaining the role of Vps1 intrans-SNARE formation. Vps1 in its polymeric state recruits multiple Qa-SNAREs to the tether HOPS. As Vps1 is bound to the SNARE domain of Vam3, it has to be released before the formation oftrans-SNAREs. After GTP hydrolysis and concomitant Vps1 release have occurred, multipletrans-SNAREs form at the fusion site. In the absence of Vps1 or in the presence of mutations in Vps1 leading to defects in GTP hydrolysis or polymerization, the number of formedtrans-SNAREs does not reach the necessary threshold at the fusion site to promote complete membrane fusion. Figure 4: Dynasore inhibits vacuolar fission and fusion in vivo . ( A ) Vacuoles of wild-type yeast cells were labelled with FM4-64 using the standard procedure as described in the Methods section. In the assay for fragmentation, (a) shows the normal vacuole structure of logarithmic phase wild-type cells, (b) shows salt-induced fragmentation of vacuoles in the presence of solvent DMSO. (c) Salt-induced phenotype of vacuoles in the presence of 100 μM dynasore. The percentage of cells showing normal or fragmented vacuoles was quantified. One hundred cells were counted randomly in each experiment. Three independent experiments are shown as means±s.d. In the assay for fusion (d) shows the fragmented vacuoles after salt exposure; (e) shows the effect of the solvent DMSO on re-fusion of fragmented vacuoles; (f) displays the influence of dynasore on re-fusion of fragmented vacuoles. The percentage of cells exhibiting normal or fragmented vacuoles was quantified. One hundred cells were counted randomly in each experiment. Three independent experiments are shown as means ±s.d. Scale bar 5 μm. ( B ) Dynasore at a concentration of 100 μM inhibits in vitro vacuole fusion and trans -SNARE complex formation. ( C ) Dynasore inhibits the GTPase activity of recombinant Vps1. ( D ) Model explaining the role of Vps1 in trans -SNARE formation. Vps1 in its polymeric state recruits multiple Q a -SNAREs to the tether HOPS. As Vps1 is bound to the SNARE domain of Vam3, it has to be released before the formation of trans -SNAREs. After GTP hydrolysis and concomitant Vps1 release have occurred, multiple trans -SNAREs form at the fusion site. In the absence of Vps1 or in the presence of mutations in Vps1 leading to defects in GTP hydrolysis or polymerization, the number of formed trans -SNAREs does not reach the necessary threshold at the fusion site to promote complete membrane fusion. Full size image We have demonstrated that Vps1 is an essential factor in vacuolar fusion. In the absence of Vps1, as well as in the presence of excess rVps1, vacuolar fusion and trans -SNARE establishment are impaired. We interpret the data as a two step process. First, Vps1 induces a population of Vam3 that associates with HOPS rather than pairing with other SNAREs. Although cis -SNARE complexes can be considered as a reservoir for single SNAREs dependent on activation through Sec18/NSF, the HOPS-associated fraction of Vam3 is likely essential for organizing SNARE nucleation and trans -SNARE formation [27] , [29] . Our data suggest that the population of HOPS-associated Vam3 is absent on vps1Δ vacuoles. As Vps1 predominantly interacts with the SNARE domain of Vam3, it prevents the formation of SNARE complexes in the initial phase of membrane fusion. Consequently, to initiate SNARE nucleation and trans -SNARE interactions, Vps1 has to be released from Vam3 [17] . Addition of excess recombinant Vps1 impairs this process and inhibits vacuolar fusion and trans -SNARE formation, emphasizing the importance of the release event. A second function of Vps1 might be the control of SNARE density with the tethering complex HOPS. Vps1 might actively increase SNARE density at the contact site of two fusing membrane by recruiting several Q a SNAREs to the tethering complex ( Fig. 4D ). Dynamin with its tendency to polymerize under the appropriate conditions and with its ability to interact with SNARE proteins is likely to be an important regulator of SNARE complex density at the fusion site. This is supported by our data showing that in the GTPase- and polymerization-deficient Vps1 mutants K42A and I649K, the amount of HOPS-associated Vam3 and extent of trans -SNARE formation is significantly lower compared with wild type. Currently, there is ample discussion about the exact number of trans -SNARE complexes needed to promote full content mixing between two fusing membranes, varying between one and four [30] . On the basis of our observations made in the I649K Vps1 mutant, we prefer the idea of multiple trans -SNARE complexes per fusion site to promote full membrane bilayer merging. Vacuole isolation Vacuoles were isolated as described previously [17] . DKY6281 and BJ3505 strains carrying tagged SNAREs were grown in Yeast extract Peptone Dextrose (YPD) at 30 °C at 225 g to optical density (OD) 600 =2 and were collected (3 min, 5,000 g ). Vacuoles were isolated through hydrolysing yeast cell walls using lyticase [31] , recombinantly expressed in Escherichia coli RSB805 (provided Dr Randy Schekman, Berkeley), and were prepared from a periplasmic supernatant. Collected cells were resuspended in reduction buffer (30 mM Tris/Cl pH 8.9, 10 mM dithiothreitol (DTT)) and incubated for 5 min at 30 °C. After collecting the cells as described above, they were resuspended in 15 ml digestion buffer (600 mM sorbitol, 50 mM K-phosphate pH 7.5 in Yeast extract Peptone (YP) medium with 0.2% glucose and 0.1 mg ml −1 lyticase preparation). After 20 min at 30 °C, cells were centrifuged (1 min 5,800 g in JLA25.5 rotor). The spheroplasts were resuspended in 2.5 ml 15% Ficoll-400 in PS buffer (10 mM PIPES/KOH Sorbitol buffer pH 6.8, 200 mM sorbitol) and 200 μl DEAE-dextran (0.4 mg ml −1 in PS). After 90 s of incubation at 30 °C, the cells were transferred to SW41 tubes and overlaid with steps of 8, 4 and 0% Ficoll-400 in PS. Cells were centrifuged for 75 min at 2 °C and 30,000 g in a SW41 rotor. Vacuole fusion In vitro vacuole fusion assay was carried out as described previously [17] . In brief, DKY6281 and BJ3505 vacuoles were adjusted to a protein concentration of 0.5 mg ml −1 and incubated in a volume of 30 μl PS buffer (10 mM PIPES/KOH pH 6.8, 200 mM sorbitol) with 125 mM KCl, 0.5 mM MnCl 2 , 1 mM DTT. Inhibitors were added before starting the fusion by addition of the ATP-regenerating system (0.25 mg ml −1 creatine kinase, 20 mM creatine phosphate, 500 μM ATP, 500 μM MgCl 2 ). After 60 min at 27 °C, or on ice, 1 ml of PS buffer was added, vacuoles were centrifuged (2 min, 20,000 g , 4 °C) and resuspended in 500 μl developing buffer (10 mM MgCl 2 , 0.2% TX-100, 250 mM TrisHCl pH 8.9, 1 mM p -nitrophenylphosphate). After 5 min at 27 °C, the reactions were stopped with 500 μl 1 M glycine pH 11.5 and the OD was measured at 400 nm. Trans -SNARE assay Vacuoles were adjusted to a protein concentration of 0.5 mg ml −1 . The total volume of one assay was 1 ml containing equal amounts of the two fusion partners in PS buffer with 125 mM KCl, 0.5 mM MnCl 2 and 1 mM DTT. Mixed vacuoles were incubated for 5 min at 27 °C in the absence of ATP. The fusion reaction was started by adding ATP-regenerating system (0.25 mg ml −1 creatine kinase, 20 mM creatine phosphate, 500 μM ATP, 500 μM MgCl 2 ). After 30 min at 27 °C, the vacuoles were centrifuged for 2 min at 4 °C at 20,000 g . The pellet was resuspended in 1.5 ml solubilization buffer (0.5% Triton, 50 mM KCl, 3 mM EDTA, 1 mM DTT in PS). After centrifugation for 4 min at 4 °C (20,000 g ), the supernatant was incubated with 30 μl Protein G beads (Roche) and 15 μg HA-antibodies (Covance, mouse monoclonal) for 1 h at 4 °C with gentle shaking. The Protein G beads were washed three times with 50 mM KCl, 0.25% Triton, 3 mM DTT and 3 mM EDTA in PS buffer, and incubated for 5 min at 60 °C in 2 × reducing SDS sample buffer. In vivo fragmentation and re-fusion assay Logarithmic grown BJ3505 cells were stained with FM4-64 (10 μM) for 30 min at 30 °C in YPD and subsequently chased for another 60 min. To visualize dynasore’s effect on fragmentation, stained cells were incubated for 1 h in YPD in the presence of 100 μM dynasore. Thereafter, cells were briefly centrifuged and further incubated in YPD supplemented with 200 mM KCl and 100 μM dynasore. After 10 min cells were inspected for fragmentation using fluorescence confocal microscopy. To investigate dynasore’s impact on fusion, stained cells were first fragmented by a brief incubation in YPD containing 400 mM KCl (10 min). Dynasore then was added at a concentration of 100 μM, and cells were incubated for a further 10 min in the high-salt YPD. Afterwards, cells were briefly centrifuged and released from the osmotic pressure by addition of normal YPD containing 100 μM dynasore. After 20 min, cells were inspected for re-fusion of fragmented vacuoles using fluorescence confocal microscopy. HOPS precipitation assay Vacuoles were isolated from BJ3505 wild-type and vps1 Δ strains harbouring Vps33-HA. Two milligram of vacuoles purified from each strain were incubated with or without ATP in PS buffer containing 100 mM KCl and 500 μM MnCl 2 for 15 min at 27 °C. Subsequently, the vacuoles were solubilized in buffer containing 100 mM KCl, 500 μM MnCl 2 and 0.3% TritonX-100. The samples were centrifuged at 20,000 g for 10 min, and 10 μg of HA antibody (Covance) and Protein G beads were added to the solubilizate. After incubation for 1 h at 4 °C with end-to-end rotation, the samples were centrifuged for 1 min and the beads were washed twice with solubilization buffer. SDS sample buffer was added to the beads and incubated at 90 °C for 2 min. The eluted proteins were separated by SDS–PAGE and analysed by western blotting with the indicated antibodies. GST-pulldown assay Nyv1, Vam3 and Vti1 were expressed as full-length proteins devoid of the transmembrane domain from pET28 vectors harbouring a poly-His tag on their N terminus. Vam7 was expressed from a pGEX vector as a N-terminally tagged GST protein. Vps1 was expressed as a full-length protein harbouring a poly-His tag on the N terminus [2] . A solution containing 2 μg each of GST-Vam7, His-Vam3, His-Vti1 and His-Nyv1 was incubated for 1 h at 4 °C, with various amounts of His-Vps1 in PS buffer with 100 mM KCl and 1 mM DTT in the presence of glutathione beads. Thereafter, samples were briefly centrifuged and washed three times using the same buffer. Following, 2 × concentrated reducing SDS sample buffer was added to the beads and precipitated proteins were analysed using SDS–PAGE and western blotting. Dot blot assay Vam3 proteins were expressed as full-length, N-terminal domain and SNARE domain from pTYB12 vector with an intein tag on the N terminus. Vam3 full-length (1–252), the N-terminal domain (1–190) and the SNARE domain (190–252) were cloned into a pTYB12 vector using Spe I and Xho I sites. Proteins were purified as recommended in the IMPACT manual (New England Biolabs). Briefly, BL21(DE3) cells transformed with the plasmid were induced at OD 600 of 0.8–1.0 with 0.5 mM isopropyl-β- D -thiogalactoside at 16 °C overnight and bound to chitin beads after cell lysis in 20 mM HEPES, 500 mM NaCl, pH 8.0. On-column cleavage was performed for 16 h at room temperature in the same buffer, with the addition of 50 mM DTT. This was dialysed with 20 mM Tris-HCl, 50 mM NaCl, pH 7.0. Vps1 was expressed as His-Vps1 was purified, as described earlier [2] . Vam3 samples (1 μg) were applied to a nitrocellulose membrane and blocked with 5% skim milk for 1 h at room temperature. Vps1 at a concentration of 10 μg ml −1 in 5% skim milk was added to the membrane and incubated overnight at 4 °C. The membrane was washed with PBS for 5 min and incubated with anti-Vps1 antibodies for 1 h at room temperature. Subsequently, the membrane was washed with PBS for 5 min and incubated with anti-rabbit secondary antibodies. GTPase assay GTP hydrolysis was followed by monitoring release of P i , which was quantified by a colorimetric method as described [32] . For basal GTPase assays, Vps1 was diluted to 1 μM in GTPase assay buffer (20 mM HEPES–KOH pH 7.5, 150 mM KCl, 2 mM MgCl 2 , 1 mM DTT). Vps1 was incubated with dynasore at a concentration of 100 μM for 20–30 min at room temperature with shaking. The inhibitor stock was freshly prepared at a final concentration of 3 mM in DMSO. GTP was added to the samples at a final concentration of 1 mM and incubated at 37 °C for 15 min with shaking. The reactions were stopped with 100 mM EDTA, pH 8.0. The free orthophosphate was measured using a malachite green phosphate assay kit (Bioassay System). Microscopy Images were taken from a Leica TCS SP5 confocal microscope using an argon laser. Images were exported as TIFF files. Images were cropped from TIFF files and pasted into Adobe Illustrator CS3. The final figure file was saved as adobe illustrator (.ai) format. Western blot images The western blot images were taken from a LI-COR Odyssey Infrared Imager. The files were exported as TIFF and processed in adobe illustrator CS3. The band intensity was quantified using densitometry software supplied with the Odyssey Infrared Imager. How to cite this article: Alpadi, K. et al. Dynamin–SNARE interactions control trans -SNARE formation in intracellular membrane fusion. Nat. Commun. 4:1704 doi: 10.1038/ncomms2724 (2013).